Essential regulation of cell bioenergetics inTrypanosoma bruceiby the mitochondrial calcium uniporter Mechanisms of regulation of mitochondrial metabolism in trypanosomes are not completely understood. Here we present evidence that the Trypanosoma brucei mitochondrial calcium uniporter ( Tb MCU) is essential for the regulation of mitochondrial bioenergetics, autophagy and cell death, even in the bloodstream forms that are devoid of a functional respiratory chain and oxidative phosphorylation. Localization studies reveal its co-localization with MitoTracker staining. TbMCU overexpression increases mitochondrial Ca 2+ accumulation in intact and permeabilized trypanosomes, generates excessive mitochondrial reactive oxygen species (ROS) and sensitizes them to apoptotic stimuli. Ablation of TbMCU in RNAi or conditional knockout trypanosomes reduces mitochondrial Ca 2+ uptake without affecting their membrane potential, increases the AMP/ATP ratio, stimulates autophagosome formation and produces marked defects in growth in vitro and infectivity in mice, revealing its essentiality in these parasites. The requirement of Tb MCU for proline and pyruvate metabolism in procyclic and bloodstream forms, respectively, reveals its role in regulation of mitochondrial bioenergetics. T rypanosoma brucei belongs to the group of parasites that causes nagana in cattle and African sleeping sickness in humans, one of the most neglected diseases in the world. Two of its life cycle stages that are easily grown in the laboratory are the procyclic form (PCF), which is one of the forms present in the tse tse fly vector, and the bloodstream form (BSF), which is present in the blood of the infected mammalian host. Each form has a single mitochondrion that greatly differs in morphology and metabolism. The PCF mitochondrion is well developed and has a respiratory chain, while the BSF mitochondrion is more rudimentary, does not possess a functional respiratory chain or oxidative phosphorylation and relies on the reverse action of the ATP synthase to maintain the mitochondrial membrane potential [1] , [2] , [3] , [4] . Proline is the key energy source within the tse tse fly [5] , [6] and probably the main energy source of the PCF [7] , [8] , [9] through the mitochondrial generation of ATP by oxidative phosphorylation [10] , [11] . In contrast, glucose is abundant in the blood of the mammalian host and the parasite has adapted to the availability of this substrate by using glycolysis as the main source of ATP, with generation of pyruvate, which is mostly excreted to maintain its intracellular pH [12] . In mammalian cells, mitochondrial Ca 2+ uptake through the mitochondrial calcium uniporter (MCU) is required to provide reducing equivalents to support oxidative phosphorylation [13] through activation of three intramitochondrial dehydrogenases [14] , [15] and the ATP synthase [16] . Interestingly, BSF possess a MCU [1] despite the absence of respiratory chain and oxidative phosphorylation [17] . The MCU has low affinity and high capacity for Ca 2+ uptake and although it was first identified more than 50 years ago [18] , [19] its molecular nature was discovered only recently [20] , [21] . Evidence of the presence of a MCU in trypanosomes [22] , [23] and its absence in yeast [24] was the key to the discovery of the molecular identity of MCU [20] , [21] , and of one modulator of the uniporter, the mitochondrial calcium uptake 1 or MICU1 (ref. 25 ), in mammalian cells [17] . Although the relevance of the MCU in mitochondrial Ca 2+ uptake has been elucidated [20] , [21] , [26] , it is not yet known whether this channel is essential for the survival of any organism. In addition, the presence of a MCU in the mitochondria of BSF, which are devoid of respiratory chain and oxidative phosphorylation, suggests that Ca 2+ could have other functions in the mitochondria of these cells. In this work, we report that knockdown of the T. brucei MCU ( TbMCU ) gene by RNA interference (RNAi) in PCF and BSF trypanosomes or by conditional knockout (KO) in BSF trypanosomes led to marked decrease in mitochondrial calcium uptake without affecting their membrane potential, and marked growth defects in vitro and reduced infectivity in vivo, underscoring the relevance of this channel for parasite survival. In addition, we demonstrate the role of the MCU in maintaining mitochondrial bioenergetics in both PCF and BSF trypanosomes. Characterization of Tb MCU One gene (Tb927.11.1350) encoding a putative MCU was found in the T. brucei genome at the TriTryp database ( http://www.tritrypdb.org/tritrypdb/ ) and named TbMCU . The full-length complementary DNA of TbMCU was cloned by PCR amplification and confirmed by sequencing as described in Methods. The orthologues identified in T. cruzi (TcCLB.503893.120) and Leishmania major (LmjF27.0780) shared 49 and 41% amino-acid identity, respectively, to TbMCU , which shares 20% identity and 33% similarity with the human MCU. Structural analysis (ELM and TMHMM servers) predicted two transmembrane domains in the carboxy-terminal region between amino acids 201–223 and 233–250. The open reading frame predicts a mature (or processed) protein of 259 amino acids with an apparent molecular weight of 30 kDa, preceded by a 48 amino acid amino-terminal mitochondrial targeting signal. A motif for the putative Ca 2+ -specific selectivity filter (WDIMEPV) is present in the loop between transmembrane domains at the C-terminal region. Tb MCU localization in PCF and BSF trypanosomes To investigate the localization of T. brucei MCU, a C-terminal green fluorescence protein (GFP)-tagged Tb MCU transgenic cell line was generated in PCF trypanosomes. Western blot analysis confirmed expression of proteins of the expected size ( Supplementary Fig. S1a ). The detection of two bands of tagged Tb MCU has been shown before when tagging the mammalian MCU [20] , [27] and could be due to interference of the tag with the processing of the N -terminal mitochondrial targeting signal, as only one band is detected when using antibodies against the protein (see below; Fig. 1h,i ). The GFP-tagged cells grew at the same rate as the wild-type cells ( Supplementary Fig. S1b ). TbMCU localized to the mitochondria, as demonstrated by co-localization with MitoTracker ( Fig. 1a ). To eliminate the possibility of mis-targeting of the GFP-tagged protein, antibodies against Tb MCU were generated through immunization of mice with the recombinant protein. The purified antibody specifically bound to the mitochondria of PCF ( Fig. 1b ) and BSF ( Fig. 1c ) trypanosomes, as shown by co-localization with MitoTracker. 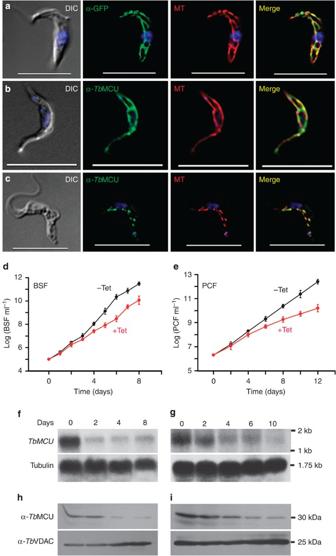Figure 1:TbMCU co-localizes with MitoTracker and its downregulation by RNAi affects growth in PCF and BSF trypanosomes. (a)TbMCU-GFP co-localization with MitoTracker (MT) in mitochondria of PCF trypanosomes as detected by immunofluorescence analyses with antibodies against GFP (Pearson’s correlation coefficient (PCC): 0.912). (b,c)TbMCU co-localization with MitoTracker in the mitochondria of PCF (b) or BSF (c) trypanosomes, as detected by immunofluorescence analyses with antibodies againstTbMCU. PCC: 0.930 and 0.920, respectively. Merge images show the co-localization in yellow. DIC, differential interference contrast microscopy. Scale bar, 10 μm (a–c). (d,e) Growth of BSF (d) and PCF (e) trypanosomes in the absence (black lines,−Tet) or presence (red lines,+Tet) of 1 μg ml−1tetracycline for the indicated number of days. Values are mean±s.d. (n=3). (f,g) Northern blot analyses ofTbMCURNAi of BSF (f) and PCF (g) trypanosomes grown in the absence (0) and presence (2–8; 2–10) of tetracycline (top). Tubulin is shown as a loading control (bottom). Markers are shown on the right. The transcript ofTbMCU, including the 5′- and 3′-UTR was ~1.5 kb in length. (h,i) Western blot analyses ofTbMCURNAi of BSF (h) and PCF (i) trypanosomes grown in the absence (0) or presence (2–8; 2–10) of tetracycline. Total lysates (30 μg) were subjected to 10% SDS–polyacrylamide gel electrophoresis before transfer to a nitrocellulose membrane and then stained with antibodies againstTbMCU (top). One band of ~30 kDa was detected inT. bruceihomogenates. Membranes were stripped and re-incubated with antibody against the voltage-dependent anion channel (TbVDAC) as a loading control (bottom). Figure 1: Tb MCU co-localizes with MitoTracker and its downregulation by RNAi affects growth in PCF and BSF trypanosomes. ( a ) Tb MCU-GFP co-localization with MitoTracker (MT) in mitochondria of PCF trypanosomes as detected by immunofluorescence analyses with antibodies against GFP (Pearson’s correlation coefficient (PCC): 0.912). ( b , c ) Tb MCU co-localization with MitoTracker in the mitochondria of PCF ( b ) or BSF ( c ) trypanosomes, as detected by immunofluorescence analyses with antibodies against Tb MCU. PCC: 0.930 and 0.920, respectively. Merge images show the co-localization in yellow. DIC, differential interference contrast microscopy. Scale bar, 10 μm ( a – c ). ( d , e ) Growth of BSF ( d ) and PCF ( e ) trypanosomes in the absence (black lines, −Tet ) or presence (red lines, +Tet ) of 1 μg ml −1 tetracycline for the indicated number of days. Values are mean±s.d. ( n =3). ( f , g ) Northern blot analyses of TbMCU RNAi of BSF ( f ) and PCF ( g ) trypanosomes grown in the absence (0) and presence (2–8; 2–10) of tetracycline (top). Tubulin is shown as a loading control (bottom). Markers are shown on the right. The transcript of TbMCU , including the 5′- and 3′-UTR was ~1.5 kb in length. ( h , i ) Western blot analyses of TbMCU RNAi of BSF ( h ) and PCF ( i ) trypanosomes grown in the absence (0) or presence (2–8; 2–10) of tetracycline. Total lysates (30 μg) were subjected to 10% SDS–polyacrylamide gel electrophoresis before transfer to a nitrocellulose membrane and then stained with antibodies against Tb MCU (top). One band of ~30 kDa was detected in T. brucei homogenates. Membranes were stripped and re-incubated with antibody against the voltage-dependent anion channel ( Tb VDAC) as a loading control (bottom). Full size image Tb MCU is required for optimal growth in vitro Knockdown of TbMCU by induction of double-stranded RNA resulted in growth defects in both BSF ( Fig. 1d ) and PCF trypanosomes ( Fig. 1e ). The effects were most pronounced with PCF trypanosomes, with up to 64±7% reduction in the number of cells at day 10, while there was a 56±6% reduction in the number of BSF trypanosomes at day 6. Northern blot and ImageJ analyses showed that the messenger RNA was downregulated by 32–75% after 4–10 days of tetracycline addition to PCF trypanosomes ( Fig. 1g ). Similar results were observed after RNAi of BSF trypanosomes ( Fig. 1f ), although the mRNA recovered from 60% at 4 days to 45% knockdown after 8 days. Western blot analyses revealed a correlative decrease in Tb MCU expression in both BSF ( Fig. 1h ) and PCF ( Fig. 1i ) trypanosomes. All further phenotypic analyses were performed on day 4 of RNAi induction for both PCF and BSF trypanosomes, unless indicated otherwise. RNAi of TbMCU reduces mitochondrial Ca 2+ uptake Mitochondrial Ca 2+ ([Ca 2+ ] m ] was significantly decreased under resting conditions in Tb MCU knockdown PCF trypanosomes ( Supplementary Fig. S1c ), while cytosolic Ca 2+ ([Ca 2+ ] i ] was not affected ( Supplementary Fig. S1d ). To determine their ability to take up Ca 2+ , we selectively permeabilized the plasma membrane of PCF trypanosomes with digitonin, as described before [1] , and monitored Ca 2+ uptake with Calcium Green-5N. 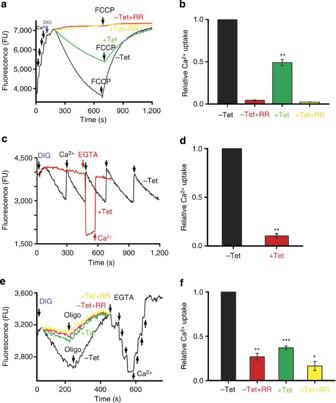Figure 2: Silencing ofTbMCUexpression decreases Ca2+uptake of digitonin-permeabilized PCF and BSF trypanosomes. (a) The reaction buffer contained 2 mM succinate and 1 μM Calcium Green 5-N. After several pulses of Ca2+(8 μM final concentration) cells (5 × 107trypanosomes grown in the absence (black tracing) or presence (green tracing) of tetracycline) were added to the reaction medium (2.45 ml) and the reaction was started adding 50 μM digitonin. Ruthenium red (RR, 40 μM, yellow and red tracing), and FCCP (5 μM) were added where indicated. A decrease in fluorescence indicates decreasing medium Ca2+or increasing vesicular Ca2+. (b) Relative Ca2+uptake at 700 s as compared with that of control trypanosomes grown in the absence of tetracycline considered as 1.0 (−Tet) (means±s.d.,n=3, **P<0.001, Student’st-test). (c) Similar conditions as inaexcept that further CaCl2additions (8 μM each time) were added to −Tettrypanosomes to show the high mitochondrial capacity to take up Ca2+. EGTA (8 μM) and CaCl2(Ca2+) were added where indicated to show the presence of medium Ca2+. (d) Relative initial rate of Ca2+uptake by +Tetas compared with −Tettrypanosomes (means±s.d.,n=3, **P<0.001, Student’st-test). (e) Representative traces of Ca2+uptake kinetics in digitonin-permeabilizedTbMCU BSFtrypanosomes cultured in the absence (−Tet) or presence (+Tet) of tetracycline. The reactions were started adding 40 μM digitonin in the presence of 1 mM ATP and 500 μM sodium orthovanadate. Ca2+uptake was monitored over time using 1 μM Calcium Green-5N. Ruthenium red (RR, 40 μM, yellow and red tracings), oligomycin (Oligo, 2.5 μg ml−1), EGTA (0.4 μM) and CaCl2(pulses of 0.4 μM) were added where indicated. (f) Relative Ca2+uptake at 200 s as compared with that of control BSF trypanosomes grown in the absence of tetracycline considered as 1 (−Tet) (means±s.d.,n=3, *(+Tet±RR), **(−Tet±RR), ***(−Tet/+Tet) ,P<0.001, Student’st-test). Figure 2a shows that when 50 μM digitonin was added to a reaction medium containing PCF trypanosomes, 2 mM succinate and 40 μM Ca 2+ , a fast decrease in Ca 2+ concentration started after a period of about 30 s and continued until addition of the uncoupler carbonyl cyanide 4-(trifluoromethoxy) phenylhydrazone (FCCP) released the Ca 2+ taken up. This Ca 2+ -transporting activity was fully abrogated by the addition of 40 μM of the MCU inhibitor ruthenium red, indicating that it is due to the MCU. Knockdown of the expression of TbMCU in PCF trypanosomes by RNAi significantly reduced their ability take up Ca 2+ , which was also abrogated by ruthenium red ( Fig. 2a,b ). The mitochondria of permeabilized control PCF trypanosomes were capable of buffering multiple pulses of exogenously added Ca 2+ ( Fig. 2c ). However, TbMCU -silenced PCF trypanosomes showed a strong attenuated response, hardly buffering a single pulse ( Fig. 2c,d ). Figure 2: Silencing of TbMCU expression decreases Ca 2+ uptake of digitonin-permeabilized PCF and BSF trypanosomes. ( a ) The reaction buffer contained 2 mM succinate and 1 μM Calcium Green 5-N. After several pulses of Ca 2+ (8 μM final concentration) cells (5 × 10 7 trypanosomes grown in the absence (black tracing) or presence (green tracing) of tetracycline) were added to the reaction medium (2.45 ml) and the reaction was started adding 50 μM digitonin. Ruthenium red (RR, 40 μM, yellow and red tracing), and FCCP (5 μM) were added where indicated. A decrease in fluorescence indicates decreasing medium Ca 2+ or increasing vesicular Ca 2+ . ( b ) Relative Ca 2+ uptake at 700 s as compared with that of control trypanosomes grown in the absence of tetracycline considered as 1.0 (− Tet ) (means±s.d., n =3, ** P <0.001, Student’s t -test). ( c ) Similar conditions as in a except that further CaCl 2 additions (8 μM each time) were added to − Tet trypanosomes to show the high mitochondrial capacity to take up Ca 2+ . EGTA (8 μM) and CaCl 2 (Ca 2+ ) were added where indicated to show the presence of medium Ca 2+ . ( d ) Relative initial rate of Ca 2+ uptake by + Tet as compared with − Tet trypanosomes (means±s.d., n =3, ** P <0.001, Student’s t -test). ( e ) Representative traces of Ca 2+ uptake kinetics in digitonin-permeabilized TbMCU BSF trypanosomes cultured in the absence (− Tet ) or presence (+ Tet ) of tetracycline. The reactions were started adding 40 μM digitonin in the presence of 1 mM ATP and 500 μM sodium orthovanadate. Ca 2+ uptake was monitored over time using 1 μM Calcium Green-5N. Ruthenium red (RR, 40 μM, yellow and red tracings), oligomycin (Oligo, 2.5 μg ml −1 ), EGTA (0.4 μM) and CaCl 2 (pulses of 0.4 μM) were added where indicated. ( f ) Relative Ca 2+ uptake at 200 s as compared with that of control BSF trypanosomes grown in the absence of tetracycline considered as 1 (− Tet ) (means±s.d., n =3, *( +Tet ± RR ), **(− Tet ± RR ), ***(− Tet/+Tet ) , P <0.001, Student’s t -test). Full size image The mitochondria of BSF trypanosomes lack cytochromes and does not have oxidative phosphorylation. Ca 2+ uptake by these mitochondria can be measured by addition of ATP in the presence of sodium orthovanadate to inhibit other non-mitochondrial Ca 2+ -ATPases ( Fig. 2e ) [1] . Ca 2+ uptake was significantly lower when the expression of TbMCU was silenced by RNAi and in both cases it was almost completely abrogated by addition of ruthenium red ( Fig. 2e,f ). Addition of oligomycin released Ca 2+ taken up, indicating the inhibition of the ATP synthase working as an ATPase [1] . Additions of EGTA and Ca 2+ shown in Fig. 2e were done to calibrate the Ca 2+ concentrations. RNAi of TbMCU does not alter membrane potential Previous work with the use of safranine determined that mitochondria in situ of PCF trypanosomes are able to build up and retain a membrane potential of the order of 140 mV [1] . 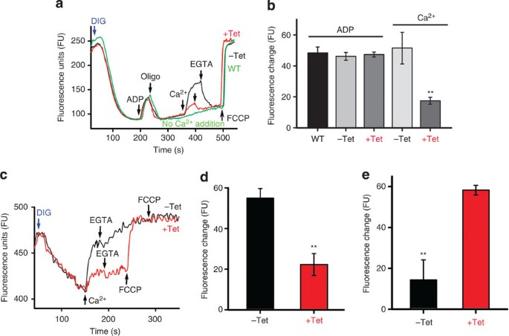Figure 3: Silencing ofTbMCUexpression does not affect the mitochondrial membrane potential of digitonin-permeabilized PCF and BSF trypanosomes. (a) PCF trypanosomes (5 × 107cells) were added to the reaction buffer (2.45 ml) containing 2 mM succinate, and 5 μM safranine, and the reaction was started with digitonin (50 μM). ADP (10 μM), oligomycin (Oligo, 2 μg ml−1), CaCl2(40 μM), EGTA (200 μM) and FCCP (10 μM) were added where indicated. (b) Changes in safranine fluorescence after addition of ADP or Ca2+to −Tetand +TetPCF trypanosomes (means±s.d.,n=3, **P<0.01, Student’st-test). (c) BSF trypanosomes (2 × 108cells) were added to the reaction buffer (2.45 ml) containing EGTA (20 μM), ATP (1 mM), sodium orthovanadate (500 μM) and 12.5 μM safranine. The reaction was started with digitonin (40 μM). CaCl2(50 μM), EGTA (200 μM) and FCCP (10 μM) were added where indicated. (d,e) Changes in safranine fluorescence after addition of Ca2+(d) or FCCP (e) to −Tetand +TetBSF trypanosomes (means±s.d.,n=3, **P<0.01, Student’st-test). Figure 3a shows that addition of ADP to these preparations was followed by the expected [28] small decrease in membrane potential that was inhibited by addition of the ATP synthase inhibitor oligomycin, indicating ADP phosphorylation. Addition of 40 μM CaCl 2 was followed by a larger decrease compatible with the electrophoretic influx of Ca 2+ into the mitochondria, which returned almost to basal levels after addition of 200 μM EGTA. Further addition of FCCP collapsed the membrane potential. Knockdown of the expression of TbMCU in PCF trypanosomes by RNAi significantly reduced the ability of their mitochondria to decrease the membrane potential because of Ca 2+ uptake, without affecting the mitochondrial membrane potential or ADP phosphorylation ( Fig. 3a,b ), indicating that only the ability of taking up Ca 2+ was affected. Figure 3: Silencing of TbMCU expression does not affect the mitochondrial membrane potential of digitonin-permeabilized PCF and BSF trypanosomes. ( a ) PCF trypanosomes (5 × 10 7 cells) were added to the reaction buffer (2.45 ml) containing 2 mM succinate, and 5 μM safranine, and the reaction was started with digitonin (50 μM). ADP (10 μM), oligomycin (Oligo, 2 μg ml −1 ), CaCl 2 (40 μM), EGTA (200 μM) and FCCP (10 μM) were added where indicated. ( b ) Changes in safranine fluorescence after addition of ADP or Ca 2+ to − Tet and + Tet PCF trypanosomes (means±s.d., n =3, ** P <0.01, Student’s t -test). (c) BSF trypanosomes (2 × 10 8 cells) were added to the reaction buffer (2.45 ml) containing EGTA (20 μM), ATP (1 mM), sodium orthovanadate (500 μM) and 12.5 μM safranine. The reaction was started with digitonin (40 μM). CaCl 2 (50 μM), EGTA (200 μM) and FCCP (10 μM) were added where indicated. ( d , e ) Changes in safranine fluorescence after addition of Ca 2+ ( d ) or FCCP ( e ) to − Tet and + Tet BSF trypanosomes (means±s.d., n =3, ** P <0.01, Student’s t -test). Full size image When safranine was added to a reaction medium containing permeabilized BSF trypanosomes in the presence of ATP and vanadate, there was a decrease in fluorescence, which indicates stacking of safranine to the energized inner mitochondrial membrane [28] . This decrease was completely reversed by oligomycin ( Supplementary Fig. S1e ) or by the protonophore FCCP ( Fig. 3c ). In contrast with the mitochondria of PCF trypanosomes ( Fig. 3a ), the decrease in ΔΨ caused by Ca 2+ was only partially reversed by EGTA probably indicating a higher sensitivity of these mitochondria to Ca 2+ damage and opening of the permeability transition pore. The decrease in ΔΨ in BSF trypanosomes, in which TbMCU was silenced by RNAi, was significantly lower than that in control cells ( Fig. 3c–e ). Phenotypic changes after RNAi of TbMCU Trypanosomes rely on amino-acid catabolism when in their insect host, with a preference for L -proline [10] . However, PCF prefer glucose when grown in medium rich in this sugar [10] . Accordingly, silencing of TbMCU in PCF trypanosomes grown in glucose-rich medium (SDM-79) had a small effect on the AMP/ATP ratio after a short incubation in glucose-rich buffer but the ratio increased more significantly in the absence of glucose ( Fig. 4a ). To investigate the relevance of the mitochondrial Ca 2+ for proline metabolism, we cultured PCF trypanosomes in glucose-depleted medium (SDM-80) [10] and found that silencing of TbMCU increased more than approximately twofold the AMP/ATP ratio of these cells ( Fig. 4b ). In agreement with these results, growth of the RNAi parasites in this medium was more strongly affected ( Supplementary Fig. 2a ) than in SDM-79 medium ( Fig. 1e ), suggesting that the decrease in ATP levels were not compatible with growth and survival. 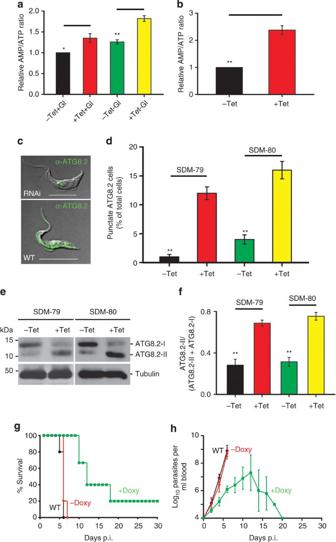Figure 4: Phenotypic changes after RNAi ofTbMCU. (a) Comparison of AMP/ATP ratios between PCF trypanosomes grown in the absence (−Tet) or presence (+Tet) of tetracycline to induce RNAi, and with or without glucose (Gl), expressed as fold increase (means±s.d.,n=3; *P<0.05; **P<0.01, Student’st-test). (b) Comparison of AMP/ATP ratios between (−Tet) and (+Tet) PCF trypanosomes grown in a glucose-depleted medium (SDM-80) containing 5.2 mML-proline for 2 days after 2-day growth in SDM-79±tetracycline, expressed as fold increase (means±s.d.,n=3, **P<0.01, Student’st-test). (c) Fluorescence microscopic images ofTbATG8.2 in PCF trypanosomes cultured in SDM-79 in the absence (WT) or presence (RNAi) of tetracycline to induce RNAi; scale bars, 10 μm. (d) Quantification of autophagosome formation in RNAi PCF trypanosomes grown in SDM-79 or SDM-80 medium in the presence (+Tet) or absence (−Tet) of tetracycline. Over 500 cells from three experiments with 20 random fields/experiment were analysed (means±s.d.,n=3, **P<0.001, Student’st-test). (e) Western blot analysis ofTbATG8.2 or tubulin in PCF trypanosomes cultured in SDM-79 or SDM-80 in the absence (−Tet) or presence (+Tet) of tetracycline to induce RNAi. Cell lysates (30 μg) were fractionated in 12% urea-SDS–PAGE gel. Immunoblots were labelled with anti-TcATG8.2 or anti-tubulin antibody. (f) Quantification of ATG8.2-II/(ATG8.2-II+ATG8.2-I) presented as mean ratios±s.d. (n=3, **P<0.01, Student’st-test). (g) Groups of five mice were infected with WTT. brucei(black line) or trypanosomes transfected with the construct for RNAi ofTbMCU(red line). Doxycycline (green line; 200 μg ml−1) was given in the drinking water throughout a 30-day period. (h) Parasitemia levels in surviving mice were monitored at 2-day intervals after infection. The results are means±s.d. (n=2). Figure 4: Phenotypic changes after RNAi of TbMCU . ( a ) Comparison of AMP/ATP ratios between PCF trypanosomes grown in the absence (− Tet ) or presence (+ Tet ) of tetracycline to induce RNAi, and with or without glucose (Gl), expressed as fold increase (means±s.d., n =3; * P <0.05; ** P <0.01, Student’s t -test). ( b ) Comparison of AMP/ATP ratios between (− Tet ) and (+ Tet ) PCF trypanosomes grown in a glucose-depleted medium (SDM-80) containing 5.2 mM L -proline for 2 days after 2-day growth in SDM-79±tetracycline, expressed as fold increase (means±s.d., n =3, ** P <0.01, Student’s t -test). ( c ) Fluorescence microscopic images of Tb ATG8.2 in PCF trypanosomes cultured in SDM-79 in the absence (WT) or presence ( RNAi ) of tetracycline to induce RNAi; scale bars, 10 μm. ( d ) Quantification of autophagosome formation in RNAi PCF trypanosomes grown in SDM-79 or SDM-80 medium in the presence ( +Tet ) or absence (− Tet ) of tetracycline. Over 500 cells from three experiments with 20 random fields/experiment were analysed (means±s.d., n =3, ** P <0.001, Student’s t -test). ( e ) Western blot analysis of Tb ATG8.2 or tubulin in PCF trypanosomes cultured in SDM-79 or SDM-80 in the absence (− Tet ) or presence (+ Tet ) of tetracycline to induce RNAi. Cell lysates (30 μg) were fractionated in 12% urea-SDS–PAGE gel. Immunoblots were labelled with anti- Tc ATG8.2 or anti-tubulin antibody. ( f ) Quantification of ATG8.2-II/(ATG8.2-II+ATG8.2-I) presented as mean ratios±s.d. ( n =3, ** P <0.01, Student’s t -test). ( g ) Groups of five mice were infected with WT T. brucei (black line) or trypanosomes transfected with the construct for RNAi of TbMCU (red line). Doxycycline (green line; 200 μg ml −1 ) was given in the drinking water throughout a 30-day period. ( h ) Parasitemia levels in surviving mice were monitored at 2-day intervals after infection. The results are means±s.d. ( n =2). Full size image Autophagy has been reported as a starvation response in different trypanosomatids (reviewed in refs 29 , 30 ), and block of mitochondrial Ca 2+ uptake by inhibitors like Ru360 in DT40 cells [13] or knockdown of MCU in HeLa cells [27] were shown to increase autophagy as a survival mechanism. In agreement with those reports, knockdown of TbMCU expression by RNAi increased the percentage of cells with autophagosomes when grown in both SDM-79 and SDM-80 media ( Fig. 4c,d ). Elevated autophagy in knockdown cells was also detected by quantitative measurements of the autophagy marker Atg8.2-II (the orthologue of LC3-II in mammalian cells) [31] ( Fig. 4e,f ). To investigate whether TbMCU is essential for the establishment of an infection in animals, we inoculated groups of five to six mice with wild type and RNAi transgenic BSF trypanosomes for TbMCU. Induction of RNAi was obtained by feeding mice with water containing doxycycline. Mice infected with the wild type and non-induced cells died 5–7 days post infection or had to be euthanized for ethical reasons when reaching parasitemias of 10 8 ml −1 ( Fig. 4g,h ). This was in contrast to the doxycycline-fed mice, where most mice survived more than 10 days. By 16 days, all, except one doxycycline-fed mice, died, suggesting that a small number of parasites (RNAi escape mutants) are able to survive in the presence of doxycycline and subsequently outgrow and kill the mice. In agreement with this suggestion, tetracycline addition in vitro reduced but did not completely eliminate the expression of TbMCU ( Fig. 1h ). Doxycycline alone is known to have no effects on mice survival under the conditions used [32] . TbMCU is essential in BSF trypanosomes Silencing of TbMCU by RNAi caused marked growth defects in vitro ( Fig. 1d,e ) and in vivo ( Fig. 4g,h ). To confirm the essentiality of TbMCU , we analysed the phenotypic changes of BSF trypanosomes with a conditional KO of the gene. In these cells, we replaced both TbMCU alleles with drug resistance genes ( Supplementary Fig. S3a–c , Supplementary Table S1 ), but, as TbMCU could be required for growth, we introduced an ectopic copy of the TbMCU gene tagged with haemagglutinin (HA), whose expression depended on the presence of tetracycline in the culture medium. Growth of the parasites in culture was greatly decreased in the absence of tetracycline and the cells died after 4–5 days of culture ( Fig. 5a ). The genotype of the mutant cell line was verified by Southern blot analysis ( Fig. 5b ). Levels of mRNA in the presence or absence of tetracycline were analysed by northern blot analysis ( Fig. 5c ). As expected, no TbMCU mRNA was detected in the absence of tetracycline for the KO cell line. In the presence of tetracycline, TbMCU mRNA level of the KO mutant was comparable to that of wild-type cells because of the ectopic gene expression. After removal of tetracycline, the expression level of ectopic Tb MCU in these mutants was confirmed by western blot ( Fig. 5d ) and immunofluorescence ( Fig. 5e ) analyses using mouse monoclonal antibodies against HA. Mitochondria of permeabilized conditional KO BSF trypanosomes obtained after 4 days in the absence of tetracycline showed a profound and complete loss of Ca 2+ uptake in response to pulses of Ca 2+ ( Fig. 5f ), while their mitochondrial membrane potential remained unaffected ( Fig. 5g–i ). In vivo studies done in mice with the conditional KOs showed higher survival of mice infected with mutant parasites, compared with controls ( Supplementary Fig. S2b,c ). Wild type and doxycycline-treated mice died by 5–7 days, while in the absence of doxycycline most mice, except two that died by day 15, survived for the duration of the experiment (30 days; Supplementary Fig. S2b ) and parasitemia was not detectable after 15 days in these surviving mice ( Supplementary Fig. S2c ). 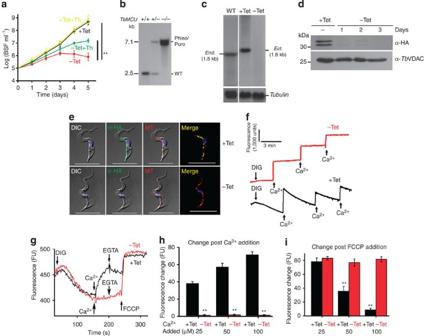Figure 5: Changes in BSF trypanosomes after conditional KO ofTbMCU. (a) Growth ofTbMCU-KO BSF in the absence (black line) or presence (red line) of 1 μg ml−1tetracycline for the indicated number of days. Addition of 10 mM threonine to the medium (green line) partially rescued the mutant BSF trypanosomes but had no effect on+Tetcells (yellow line; means±s.d.,n=3, **P<0.001, Student’st-test). (b) Southern blot analysis of the BSF conditional KOs. Genomic DNA from theT. bruceiSM parental strain (+/+), single- (+/−) or double-allele (−/−) KO cells. (c) Northern blot analysis of wild-type (WT) andTbMCU-KO BSF cultured in the presence (+Tet) or absence (−Tet) of tetracycline for 2 days. Tubulin is shown as a loading control (bottom panel). (d) Western blot analysis of total cell lysates. Proteins from BSF trypanosomes cultured in the presence(+Tet) or absence (−Tet) of tetracycline were detected using anti-HA antibody. TbVDAC was used as a loading control. (e) Immunofluorescence analysis of control (upper panels) andTbMCU-KO (lower panels) trypanosomes.TbMCU co-localized with MitoTracker (MT) in the control parasites (+Tet; PCC=0.808). Scale bar, 10 μm. (f) ConditionalTbMCU-KO BSF trypanosomes were grown in the presence (+Tet) or absence (−Tet) of tetracycline for 2 days. BSF trypanosomes (2 × 108cells) were incubated as inFig. 2e. Multiple pulses of CaCl2(arrowheads) were added to a final concentration of 20 μM. A representative trace (red or black) of Ca2+uptake from one of three independent experiments is shown. (g) Representative traces of mitochondrial membrane potential of digitonin-permeabilized BSF trypanosomes grown in the presence (+Tet) or absence (−Tet) of tetracycline. The reactions were incubated as inFig. 3c. CaCl2(50 μM), EGTA (200 μM) and FCCP (10 μM) were added where indicated. (h,i) Changes in safranine fluorescence after addition of Ca2+(h, as ing, but 25, 50 and 100 μM CaCl2) or FCCP (i) to +Tetand −TetBSF trypanosomes (means±s.d.,n=3, **P<0.001, Student’st-test). Figure 5: Changes in BSF trypanosomes after conditional KO of TbMCU . ( a ) Growth of TbMCU- KO BSF in the absence (black line) or presence (red line) of 1 μg ml −1 tetracycline for the indicated number of days. Addition of 10 mM threonine to the medium (green line) partially rescued the mutant BSF trypanosomes but had no effect on +Tet cells (yellow line; means±s.d., n =3, ** P <0.001, Student’s t -test). ( b ) Southern blot analysis of the BSF conditional KOs. Genomic DNA from the T. brucei SM parental strain (+/+), single- (+/−) or double-allele (−/−) KO cells. ( c ) Northern blot analysis of wild-type (WT) and TbMCU -KO BSF cultured in the presence ( +Tet ) or absence (− Tet ) of tetracycline for 2 days. Tubulin is shown as a loading control (bottom panel). ( d ) Western blot analysis of total cell lysates. Proteins from BSF trypanosomes cultured in the presence (+Tet ) or absence (− Tet ) of tetracycline were detected using anti-HA antibody. TbVDAC was used as a loading control. ( e ) Immunofluorescence analysis of control (upper panels) and TbMCU -KO (lower panels) trypanosomes. Tb MCU co-localized with MitoTracker ( MT ) in the control parasites ( +Tet ; PCC=0.808). Scale bar, 10 μm. ( f ) Conditional TbMCU -KO BSF trypanosomes were grown in the presence (+ Tet ) or absence (− Tet ) of tetracycline for 2 days. BSF trypanosomes (2 × 10 8 cells) were incubated as in Fig. 2e . Multiple pulses of CaCl 2 (arrowheads) were added to a final concentration of 20 μM. A representative trace (red or black) of Ca 2+ uptake from one of three independent experiments is shown. ( g ) Representative traces of mitochondrial membrane potential of digitonin-permeabilized BSF trypanosomes grown in the presence (+ Tet ) or absence (− Tet ) of tetracycline. The reactions were incubated as in Fig. 3c . CaCl 2 (50 μM), EGTA (200 μM) and FCCP (10 μM) were added where indicated. ( h , i ) Changes in safranine fluorescence after addition of Ca 2+ ( h , as in g , but 25, 50 and 100 μM CaCl 2 ) or FCCP ( i ) to + Tet and − Tet BSF trypanosomes (means±s.d., n =3, ** P <0.001, Student’s t -test). Full size image Although none of the dehydrogenases (pyruvate dehydrogenases (PDHs)) stimulated by Ca 2+ in vertebrates have been studied in detail in trypanosomatids [17] , the PDH E1α subunit seems to possess phosphorylation sites with similarity to those of the mammalian enzyme [33] , suggesting that, as the mammalian enzyme, it could be activated by Ca 2+ -stimulated dephosphorylation. Generation of acetyl-coenzyme A (acetyl-CoA) by the PDH is required for the formation of mitochondrial acetate, which translocates to the cytosol and is used for fatty-acid synthesis [34] , a process that is required for efficient mouse infections by BSF trypanosomes [35] . Acetyl-CoA is also used for mitochondrial fatty-acid synthesis through a FAS II pathway, which is also essential in BSF trypanosomes [36] . In this regard, we were able to detect PDH activity in BSF trypanosome lysates, although at lower levels than in PCF trypanosomes ( Supplementary Fig. S2d ). T. brucei possess a threonine dehydrogenase [37] that can also produce acetyl-CoA bypassing the need of PDH and presumably without a mitochondrial Ca 2+ requirement. In agreement with this hypothesis, addition of 10 mM threonine to the culture medium could partially rescue the BSF trypanosome mutants ( Fig. 5a ). Overexpression of Tb MCU increases oxidative stress Overexpressed TbMCU was also localized to the mitochondria of PCF trypanosomes as detected by its co-localization with MitoTracker ( Supplementary Fig. S2e,f ). Mitochondrial ( Fig. 6a,b ) but not cytosolic Ca 2+ ( Fig. 6c ) was constitutively elevated under resting conditions in TbMCU -overexpressing PCF trypanosomes. In agreement with these results, overexpression of TbMCU increased the ability of their mitochondria to accumulate Ca 2+ in response to Ca 2+ pulses ( Fig. 6d,e ), without affecting the mitochondrial membrane potential ( Fig. 6f,g ). 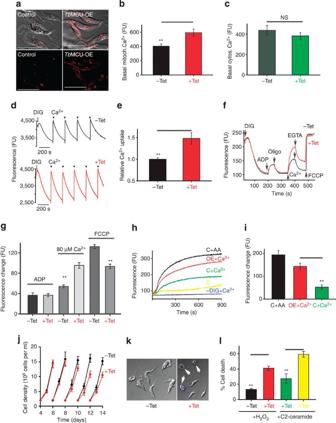Figure 6: Changes on overexpression ofTbMCU. (a) Rhod-2 fluorescence in control or overexpressingTbMCU(TbMCU-OE) PCF. Scale bar, 10 μm. (b,c) Rhod-2 (mitochondrial) (b) and Fluo-4 (cytosolic) (c) fluorescence in control (−Tet) and overexpressingTbMCU(+Tet) PCF (means±s.d.,n=3, **P<0.05, Student’st-test); NS, not significant. (d) Ca2+uptake by digitonin-permeabilized PCF overexpressingTbMCU. Trypanosomes were incubated as inFig. 2c. Multiple pulses of CaCl2(arrowheads) were added to a final concentration of 8 μM. (e) Ca2+uptake inTbMCU-OE PCF (+Tet) 200 s after addition of Ca2+, as compared with uninduced trypanosomes considered as 1 (−Tet) (means±s.d.,n=3, **P<0.01, Student’st-test). (f) Mitochondrial membrane potential of digitonin-permeabilized control (−Tet) andTbMCU-OE (+Tet) PCF. The reactions were incubated as inFig. 3a. (g) Changes in safranine fluorescence after addition of ADP, Ca2+or FCCP to–Tetand+TetPCF trypanosomes (means±s.d.,n=3, **P<0.001, Student’st-test). (h) Mitochondrial oxidative stress as measured with MitoSOX Red in control (C) andTbMCU-overexpressing (OE) PCF permeabilized with 50 μM digitonin in the presence of 0.4 mM Ca2+. Controls were treated with 2 μM antimycin A (C+AA), or were trypanosomes exposed to 0.4 mM Ca2+in the absence of digitonin (−DIG+Ca2+), and trypanosomes permeabilized with digitonin in the absence of Ca2+(C, yellow line). (i) Quantification of change at 900 s. Results are expressed as mean fluorescence±s.d. (n=3, **P<0.001, Student’st-test). (j) Growth of trypanosomes in the absence (control, black lines) or presence (TbMCU-OE, red lines) of 1 μg ml−1tetracycline (means±s.d.,n=3). (k) Dead cells in representative fields of control (−Tet) andTbMCU-OE (+Tet) PCF are indicated (white arrows). Scale bar, 10 μm. (l) Cell viability on apoptotic challenge of control (−Tet) orTbMCU-OE (+Tet) PCF trypanosomes with H2O2and C2-ceramide. The percentage of cell death was obtained from means±s.d. by analysing >60 fields (including >400 cells) (n=3). **P<0.01, Student’st-test. Figure 6: Changes on overexpression of TbMCU . ( a ) Rhod-2 fluorescence in control or overexpressing TbMCU ( TbMCU-OE ) PCF. Scale bar, 10 μm. ( b , c ) Rhod-2 (mitochondrial) ( b ) and Fluo-4 (cytosolic) ( c ) fluorescence in control (− Tet ) and overexpressing TbMCU (+ Tet ) PCF (means±s.d., n =3, ** P <0.05, Student’s t -test); NS, not significant. ( d ) Ca 2+ uptake by digitonin-permeabilized PCF overexpressing TbMCU . Trypanosomes were incubated as in Fig. 2c . Multiple pulses of CaCl 2 (arrowheads) were added to a final concentration of 8 μM. ( e ) Ca 2+ uptake in TbMCU -OE PCF (+ Tet ) 200 s after addition of Ca 2+ , as compared with uninduced trypanosomes considered as 1 (− Tet ) (means±s.d., n =3, ** P <0.01, Student’s t -test). ( f ) Mitochondrial membrane potential of digitonin-permeabilized control (− Tet ) and TbMCU -OE (+ Tet ) PCF. The reactions were incubated as in Fig. 3a . ( g ) Changes in safranine fluorescence after addition of ADP, Ca 2+ or FCCP to –Tet and +Tet PCF trypanosomes (means±s.d., n =3, ** P <0.001, Student’s t -test). ( h ) Mitochondrial oxidative stress as measured with MitoSOX Red in control (C) and TbMCU -overexpressing (OE) PCF permeabilized with 50 μM digitonin in the presence of 0.4 mM Ca 2+ . Controls were treated with 2 μM antimycin A ( C+AA ), or were trypanosomes exposed to 0.4 mM Ca 2+ in the absence of digitonin ( − DIG+Ca 2+ ), and trypanosomes permeabilized with digitonin in the absence of Ca 2+ (C, yellow line). ( i ) Quantification of change at 900 s. Results are expressed as mean fluorescence±s.d. ( n =3, ** P <0.001, Student’s t -test). ( j ) Growth of trypanosomes in the absence (control, black lines) or presence ( TbMCU-OE , red lines) of 1 μg ml −1 tetracycline (means±s.d., n =3). ( k ) Dead cells in representative fields of control (− Tet ) and TbMCU -OE (+ Tet ) PCF are indicated (white arrows). Scale bar, 10 μm. ( l ) Cell viability on apoptotic challenge of control (− Tet ) or TbMCU -OE (+ Tet ) PCF trypanosomes with H 2 O 2 and C2-ceramide. The percentage of cell death was obtained from means±s.d. by analysing >60 fields (including >400 cells) ( n =3). ** P <0.01, Student’s t -test. Full size image Mitochondrial Ca 2+ overload is known to generate oxidative stress and sensitize cells to apoptotic stimuli. Accordingly, ROS generation was increased in TbMCU -overexpressing PCF trypanosomes as compared with control cells and to comparable levels to those produced by antimycin A addition ( Fig. 6h,i ). Growth in rich medium was slightly affected by overexpression of TbMCU ( Fig. 6j ). However, overexpression of TbMCU sensitized PCF trypanosomes to apoptopic challenge. Microscopy counts of cell viability after treatment with C2-ceramide or H 2 O 2 showed that TbMCU -overexpressing trypanosomes were more efficiently killed ( Fig. 6k,l ), in agreement with the notion that mitochondrial Ca 2+ loading synergizes with apoptotic stimuli [38] , [39] . The most significant finding of our studies is that the MCU is essential in BSF trypanosomes, which are organisms devoid of oxidative phosphorylation. This pathway has been reported to be the main target of intramitochondrial Ca 2+ in vertebrate cells [13] , [14] , [15] , [16] . The partial rescue by threonine of the lethal effect of the TbMCU -KO suggests that, in contrast to what occurs in vertebrate cells, Tb MCU in BSF trypanosomes appears necessary for the generation of acetyl-CoA, not as a substrate of the Krebs cycle (tricarboxylic acid cycle) that is absent but, as either a source of intramitochondrial ATP through substrate level phosphorylation, needed for intramitochondrial anabolic reactions [40] or maintenance of the membrane potential by the ATPase [1] , or for mitochondrial [36] and/or cytosolic fatty-acid synthesis [41] . The current metabolic model in BSF trypanosomes excludes a role of the mitochondrion in the cellular provision of ATP [40] , [42] . BSF trypanosomes appear to rely exclusively on glycolysis, with cytosolic generation of ATP and excretion of pyruvate [43] . However, our results indicate that some Ca 2+ -stimulated PDH activity is present in their mitochondria and that dephosphorylation of PDH E1 α subunit (E1α) is activated by Ca 2+ , as occurs in vertebrate mitochondria. In addition to our detection of PDH activity in lysates of BSF trypanosomes, recent proteomic studies have detected the presence of not only PDH E1α and E1β (ref. 44 ) but also of the PDH E2 and E3 subunits [45] , [46] . An orthologue of the PDH phosphatase that activates the PDH E1α subunit (Tb927.5.1660) was also identified [46] . Studies of purified PDH from the bovine kidney and heart mitochondria [47] and pig heart mitochondria [48] have identified the Ser-5 of the PDH E1α sequence: Tyr-His-Gly-His- Ser -Met-Ser-Asn-Pro-Gly-Val-Ser-Tyr-Arg, as the site responsible for inactivation by phosphorylation by their intrinsic kinase. A similar peptide Tyr-Met-Gly-His- Ser -Met-Ser-Asp-Pro-Asp-Ser-Gln-Tyr-Arg is present in the T. brucei (Tb927.10.12700) orthologue. The presence of this specific serine residue in the T. brucei PDH could account for a phosphorylation/dephosphorylation model resembling mammalian E1α. The threonine dehydrogenase reaction would bypass the need of a Ca 2+ -stimulated step in the mutant parasites. Acetyl-CoA generated from pyruvate in the reaction catalysed by PDH is converted to acetate by the acetate:succinate CoA-transferase [49] or by an acetyl-CoA thioesterase [34] in PCF trypanosomes. Acetate:succinate CoA-transferase transfers the CoA group of acetyl-CoA to succinate to form succinyl-CoA, which is consequently converted back to succinate by succinyl-CoA synthase with a net production of one molecule of ATP per molecule of acetyl-CoA [34] , [49] . ATP generated by this reaction, if it occurs in BSF, or alternatively, incorporated from the cytosol by the recently described ADP/ATP carrier Tb MCP5 that is also present in BSF trypanosomes [50] , could be used for intramitochondrial metabolic reactions or for the ATPase to maintain the membrane potential. Acetate formed could then be transferred to the cytosol where is converted back into acetyl-CoA by acetyl-Co synthetase and can be used for fatty-acid synthesis [34] . Cytosolic fatty-acid synthesis appears to be essential when the BSF trypanosomes are in their mammalian host [35] despite their non-essentiality under culture conditions [41] . Alternatively, acetyl-CoA could be used for mitochondrial fatty-acid synthesis, which is known to result in the generation of lipoic acid and myristic acid, a pathway that is essential in BSF trypanosomes [36] . 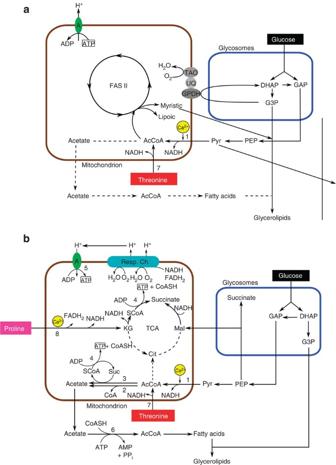Figure 7: Energy metabolism inT. brucei. Scheme of metabolic pathways in BSF (a) and PCF (b) trypanosomes. Arrows indicate steps of glucose, proline and threonine metabolism and glycerolipid biosynthesis; dashed arrows indicate steps for which no evidence of flux is available34. A, ATPase (a) or ATP synthase (b); AcCoA, acetyl-CoA; Cit, citrate, CoASH, CoA; DHAP, dihydroxyacetone phosphate; FAS II, type II fatty-acid biosynthesis pathway; GAP, glyceraldehyde 3-phosphate; G3P, glycerol 3-phosphate; GPDH, glycerol 3-phosphate dehydrogenase; KG, 2-ketoglutarate; Mal, malate; PEP, phosphoenolpyruvate; Pyr, pyruvate; Resp. Ch., respiratory chain; TCA, tricarboxylic acid cycle; UQ, ubiquinone. Enzymes are: 1, pyruvate dehydrogenase; 2, acetyl-CoA thioesterase; 3, acetate:succinate CoA-transferase; 4, succinyl-CoA synthetase; 5, F0F1-ATP synthase; 6, acetyl-CoA synthetase; TAO, trypanosome alternative oxidase; 7, threonine dehydrogenase; 8, proline dehydrogenase. Activities potentially stimulated by Ca2+are indicated. Figure 7a shows a scheme of these reactions occurring in BSF trypanosomes. Figure 7: Energy metabolism in T. brucei . Scheme of metabolic pathways in BSF ( a ) and PCF ( b ) trypanosomes. Arrows indicate steps of glucose, proline and threonine metabolism and glycerolipid biosynthesis; dashed arrows indicate steps for which no evidence of flux is available [34] . A, ATPase ( a ) or ATP synthase ( b ); AcCoA, acetyl-CoA; Cit, citrate, CoASH, CoA; DHAP, dihydroxyacetone phosphate; FAS II, type II fatty-acid biosynthesis pathway; GAP, glyceraldehyde 3-phosphate; G3P, glycerol 3-phosphate; GPDH, glycerol 3-phosphate dehydrogenase; KG, 2-ketoglutarate; Mal, malate; PEP, phosphoenolpyruvate; Pyr, pyruvate; Resp. Ch., respiratory chain; TCA, tricarboxylic acid cycle; UQ, ubiquinone. Enzymes are: 1, pyruvate dehydrogenase; 2, acetyl-CoA thioesterase; 3, acetate:succinate CoA-transferase; 4, succinyl-CoA synthetase; 5, F 0 F 1 -ATP synthase; 6, acetyl-CoA synthetase; TAO, trypanosome alternative oxidase; 7, threonine dehydrogenase; 8, proline dehydrogenase. Activities potentially stimulated by Ca 2+ are indicated. Full size image Similar to what occurs in vertebrate cells, and in contrast to what occurs in BSF trypanosomes, reduction of mitochondrial Ca 2+ transport in PCF trypanosomes in a glucose-depleted environment, or when proline is used as substrate, resulted in an increased AMP/ATP ratio. It has been demonstrated [51] that in a glucose-depleted environment, conditions present in the insect vector, PCF trypanosomes increase the rate of proline consumption and are more sensitive to oligomycin supporting the view that oxidative phosphorylation becomes essential. Proline is oxidized to glutamate through two mitochondrial steps. The first catalysed by proline dehydrogenase or proline oxidase oxidizes L -proline to Δ1-pyrroline-5-carboxylate, which is further hydrolyzed non-enzymatically to glutamic acid gamma semialdehyde. In a second enzymatic step, Δ1-pyrroline-5-carboxylate is oxidized to L -glutamate by Δ1-pyrroline-5-carboxylate dehydrogenase. Glutamate can be deaminated by transaminases or dehydrogenases to be converted into α-ketoglutarate, which through some of the Krebs cycle reactions is converted into succinate. Interestingly, the first enzyme in the proline metabolic pathway, proline dehydrogenase (Tb927.7.210), possesses an EF-hand domain and it is possibly the target for intramitochondrial Ca 2+ under these conditions. Figure 7b shows the possible reactions occurring in PCF trypanosomes. Downregulation of TbMCU in PCF trypanosomes resulted in increased autophagy, as it has also been reported when MCU was downregulated in mammalian cells [27] . It has been reported [31] that autophagy has a role in PCF trypanosomes death, although it can also be considered as a survival mechanism [13] . Although the percentage of cells with autophagosomes increased by 33% in cells grown in SDM-80, as compared with cells grown in SDM-79 medium, the difference was not significant ( P =0.065, Student’s t -test). It is known that the breakdown products derived from autophagy have a dual role providing substrates for both energy generation and biosynthesis [52] . Although we cannot rule out other mechanisms, one possible explanation for the lack of difference is that the autophagic process requires energy, for example, for the activity of the different kinases involved as well as for the synthesis/incorporation of the phagosomal membrane components [52] . Most of the products of autophagy such as amino acids and lipids yield ATP through oxidative phosphorylation [52] , which would be deficient in the absence of Tb MCU, while glycogen reserves are absent in trypanosomatids. The considerable increase in the AMP/ATP ratio in cells grown in proline-rich medium (SDM-80) in the absence of oxidative phosphorylation would prevent an increase in autophagosome formation over the level observed in cells grown in glucose-rich medium (SDM-79). Overexpression of TbMCU in PCF trypanosomes increased the ability of their mitochondria to take up Ca 2+ , resulting in mitochondrial Ca 2+ overload, oxidative stress and higher sensitivity of these mutants to proapoptotic stimuli. These results are in agreement with the results obtained after overexpression of MCU in HeLa cells [21] . However, other authors [20] did not detect marked gain of mitochondrial Ca 2+ uptake in HeLa cells overexpressing MCU . The role of mitochondrial Ca 2+ in activation of programmed cell death in mammalian cells is well recognized [53] , [54] . Mitochondrial Ca 2+ has also been recognized as important for apoptosis-like or programmed cell death in trypanosomatids. Mitochondrial Ca 2+ overload on different triggers of cell death results in ROS generation and release of cytochrome c [55] . The production of ROS in T. brucei impairs mitochondrial Ca 2+ transport, and leads to its accumulation in the nucleus and cell death [56] . T. cruzi is highly resistant to the mitochondrial permeability transition [22] , and apoptosis-like death on mitochondrial Ca 2+ overload is apparently dependent on ROS generation [57] . In vertebrate cells, mitochondrial Ca 2+ is important not only for the regulation of cellular ATP concentration but also for shaping Ca 2+ signals [58] , [59] , [60] . It is well established, through experiments using aequorin targeted to the mitochondria of T. brucei that, as in vertebrate cells, intramitochondrial Ca 2+ concentrations in T. brucei can reach values much higher than cytosolic Ca 2+ rises when Ca 2+ influx through the plasma membrane or Ca 2+ release from acidic calcium stores (acidocalcisomes) are stimulated [61] . These results suggest a very close proximity of the sole mitochondrion of the parasites with the plasma membrane and acidocalcisomes and the presence of microdomains of high Ca 2+ concentration in their vicinity. The recent finding of an inositol 1,4,5-trisphosphate (IP 3 ) receptor in acidocalcisomes of T. brucei [62] and of a close proximity of acidocalcisomes and the mitochondria in trypanosomatids [63] are compatible with a role of IP 3 -stimulated Ca 2+ release from acidocalcisomes and mitochondrial Ca 2+ uptake as a requirement for efficient mitochondrial metabolism and normal cell bioenergetics, as it has been described for the endoplasmic reticulum and mitochondria of vertebrate cells [13] . In this regard, Tb IP 3 R was found to be essential even in BSF trypanosomes [62] . One of the main functions of the MCU in trypanosomes would be, as in vertebrate mitochondria, to shape the amplitude and spatiotemporal patterns of cytosolic Ca 2+ increases [17] . In summary, our results indicate for the first time that the MCU is essential for the survival of a eukaryotic organism. In contrast to what has been recently described in some mammalian cells, where transient receptor potential 3 channels also regulate mitochondrial Ca 2+ uptake [64] , Tb MCU is the sole transporter responsible for mitochondrial Ca 2+ uptake in T. brucei . This channel is essential for growth in vitro and in vivo , and has important roles in the regulation of the cell bioenergetics in the two main life stages investigated. Reagents The p2T7 Ti vector [65] was a gift from Dr. John Donelson (University of Iowa). Rabbit polyclonal antibody against Tc ATG8.2 was a gift from Dr Vanina Alvarez (Universidad Nacional de San Martin, Argentina). Rabbit polyclonal antibody against Tb VDAC was a gift from Dr. Minu Chaudhuri (Meharry Medical College, TN). Other reagents used are described in Supplementary Methods . Culture methods T. brucei PCF (wild type and 29–13 strains) and BSF (wild type and single marker (SM) strains) were used. PCF 29–13 ( T7RNAP NEO TETR HYG ) co-expressing T7 RNA polymerase and Tet repressor were a gift from Dr George A.M. Cross (Rockefeller University, NY) and were grown in SDM-79 medium [66] supplemented with haemin (7.5 μg ml −1 ) and 10% heat-inactivated fetal bovine serum and at 27 °C in the presence of G418 (15 μg ml −1 ) and hygromycin (50 μg ml −1 ) to maintain the integrated genes for T7 RNA polymerase and tetracycline repressor, respectively. BSF (SM strain) were also a gift from Dr. G.A.M. Cross and were grown at 37 °C in HMI-9 medium [66] supplemented with 10% fetal bovine serum, 10% serum plus (JRH Biosciences, Inc.) and 2.5 μg ml −1 G418. Anti- Tb MCU antibodies The cDNA fragment of TbMCU corresponding to amino acids 49–200 was amplified by PCR and cloned in frame into the expression vector pET32 EK/Lic (Novagen) to generate pET32- TbMCU . The correct plasmid pET32- TbMCU was confirmed by sequencing and then transformed into Escherichia coli OverExpress C43 (DE3) strain (Lucigen, WI). His-tagged TbMCU fusion protein was affinity purified with Ni-NTA agarose (Qiagen) based on the manufacturer’s protocol. The purified protein was used to immunize mice and polyclonal antibodies were purified from anti-serum with Protein G Agarose Resins (Qiagen). The animal protocol was approved by the Animal Care and Use Committee of the University of Georgia. Western blot analyses The blots were incubated with mouse antibodies against Tb MCU (1:500), rabbit antibodies against GFP (1:10,000), mouse antibodies against HA (1:2,500), rabbit antibodies against Tc ATG8.2 (1:1,000), rabbit antibodies against Tb VDAC (1:2,000) or rabbit antibodies against tubulin (1:20,000) for 1 h. After five washings with PBS-T, the blots were incubated with horseradish peroxidase-conjugated anti-mouse or anti-rabbit IgG (H+L) antibody at a dilution of 1:20,000 for 1 h. After washing five times with PBS-T, the immunoblots were visualized using Pierce ECL western blotting substrate according to the manufacturer’s instructions. Full-length images of gels and immunoblots are shown in Supplementary Fig. S4 . TbMCU RNAi constructs To knockdown the expression of the TbMCU gene (Tb927.11.1350) by double-stranded RNA expression, the inducible T7 RNA polymerase-based protein expression system and the p2T7 Ti vector with dual-inducible T7 promoters were employed. A 921-bp cDNA fragment of TbMCU (targeted to the nucleotides 4–924 of the open reading frame) was amplified using the forward primer 5′-CCC AAGCTT TGGAGGCCTTATACTTTG-3′ and the reverse primer 5′-CG GGATCC TCAGTGATGTTTAAACCACTTCCG-3′ (where the underlined nucleotides indicate the introduced Bam HI and Hin dIII sites, respectively) digested with Bam HI and Hin dIII, and then cloned into the enzyme-cut p2T7 Ti vector to generate p2T7( TbMCU ). The recombinant construct p2T7( TbMCU ) was confirmed by sequencing at the DNA Analysis Facility at Yale University (New Haven, CT), Not I-linearized, and then purified with QIAGEN’s DNA purification kit for cell transfections. TbMCU has a novel nucleotide sequence without homologues (>20 nucleotide identity) in T. brucei genome/transcript databases (TriTrypDB), suggesting the absence of any other potential gene targets. Cell transfections are described in Supplementary Methods . GFP-tagged or HA-tagged Tb MCUs To construct C-terminally enhanced GFP-tagged Tb MCU for localization of Tb MCU in T. brucei , the full-length cDNA of TbMCU was amplified from T. brucei genomic DNA by PCR using the forward primer 5′-CCC AAGCTT ATGTGGAGGCCTTATACTTTG-3′ and the reverse primer 5′-CCG CTCGAG GTGATGTTTAAACCACTTCCG-3′ (where the underlined nucleotides indicate the introduced Hin dIII and Xho I sites, respectively). The PCR product was digested with Hin dIII and Xho I and then cloned in frame into the insertion sites of TbVTC1 in the pUB39 ( TbVTC1-GFP ) vector [66] to replace TbVTC1 and thus generate pUB39( TbMCU-GFP ). To construct C-terminally HA-tagged Tb MCU for overexpression or conditional KO of Tb MCU in BSF as described below, the full-length cDNA of TbMCU (924 bp) was amplified with Pfu Ultra HF DNA polymerase (Agilent) from T. brucei genomic DNA by PCR using the forward primer 5′-CCC AAGCTT ATGTGGAGGCCTTATACTTTG-3′ and the reverse primer 5′CG GGATCC CT ATG CGTAATCGGGCACATCGTACGGGTATGCGTAGTCGGGCACGTCGTATGGGTACGCGTAAT CAGGCACATCGTAAGGGTA GTGATGTTTAAACCATTCCG-3′ (where the underlined nucleotides indicate the introduced Hin dIII and Bam HI sites, respectively, and where the italicized nucleotides indicate 3 × HA-coding sequence in the reverse primer), and then cloned into the enzyme-cut pLew100v5_bsd vector to generate pLew100( TbMCU-HA ). The double-stranded sequences of GFP-tagged Tb MCU in the expression vector pUB39 and HA-tagged TbMCU in the expression vector pLew100v5_bsd were confirmed by sequencing as indicated above. The correct constructs pUB39( TbMCU-GFP ) and pLew100( TbMCU-HA ) with the inducible T7 RNA polymerase-based protein expression system were linearized by Not I and transfected into T. brucei PCF 29–13 or BSF SM trypanosomes. Northern and Southern blot analyses The TbMCU probe was generated from p2T7( TbMCU ), by PCR using the same primers described in the text, and labelled with [α- 32 P]-dCTP using a Prime-a-Gene Labeling System according to the manufacturer’s protocol. The [α- 32 P]-dCTP-labelled probe of Tb β -tubulin gene (GeneDB Tb927.1.2390) was generated from T. brucei genomic DNA by PCR using the gene-specific primers (5′-ATGCGCGAAAATCGTCTGCGTTCAGG-3′ and 5′-AGTGCAGACGCGGGAATGGGACAAG-3′). For Southern blot analysis, 10 μg Cla I-digested genomic DNA was separated on a 0.8% agarose gel and transferred to a Zeta-Probe nylon membrane. The membrane was probed with a 295-bp 32 P-labelled PCR product of the TbMCU 3′-untranslated region (UTR; Supplementary Fig. S3 ) generated with the Prime-a-Gene Labeling System. The RNA- or DNA-bound membranes were hybridized with the 32 P-labelled TbMCU or Tb β -tubulin probe in 0.5 M Na 2 HPO 4 , pH 7.4 and 7% SDS at 65 °C overnight with agitation. After hybridization, the membranes were washed twice for 10 min each at 68 °C with 1 × SSC and 0.1% SDS and then twice for 30 min at 65 °C with 0.1 × SSC and 0.1% SDS. The hybridized blots were visualized by autoradiography. Immunofluorescence microscopy To determine the localization and expression of Tb MCU in T. brucei , trypanosome live cells were labelled for 30 min with Mitotracker Red CMXRos (Invitrogen) at 50 nM in trypanosome culture medium. Bloodstream trypanosomes were washed in ice-cold PBS with 1% glucose and fixed with 1% paraformaldehyde in PBS at 4 °C for 1 h. Procyclic trypanosomes were washed with PBS and then fixed with 4% paraformaldehyde in PBS at room temperature for 1 h. The fixed parasites were washed twice with PBS, allowed to adhere to poly- L -lysine-coated coverslips and permeabilized with 0.3% Triton X-100/PBS for 3 min for PCF or 0.1% Triton X-100/PBS for 5 min for BSF. After blocking with PBS containing 3% BSA, 1% fish gelatin, 50 mM NH 4 Cl and 5% goat serum for 1 h, trypanosomes were stained in 3% BSA/PBS with the purified HA.11 clone 16B12 monoclonal antibody against HA (1:250), rabbit polyclonal antibody against GFP (1:1,000), rabbit polyclonal antibody against Tc ATG8.2 (1:250) or mouse polyclonal antibody against Tb MCU (1:50) for 1 h. After thoroughly washing with PBS containing 3% BSA, cells were incubated with Alexa 488-conjugated goat anti-mouse or anti-rabbit antibody at 1:1,000 for 1 h. The cells were counterstained with 4′,6-diamidino-2-phenylindole before mounting with Gold ProLong Gold antifade reagent (Molecular Probes). Differential interference contrast and fluorescent optical images were captured using an Olympus IX-71 inverted fluorescence microscope with a Photometrix CoolSnap HQ charge-coupled device camera driven by DeltaVision software (Applied Precision, Seattle, WA). Images were deconvolved for 15 cycles using Softwarx deconvolution software. Pearson’s correlation coefficients were calculated using the Softwarx software by measuring the whole-cell images. TbMCU conditional KO mutants To replace the endogenous TbMCU genes, phleomycin- and puromycin-resistance gene cassettes were generated by PCR amplification using the plasmids p2T7 Ti and pMOTag2T as templates with the gene-specific primers, which were designed to bind the 5′- and 3′-termini of the resistance genes followed by 149-bp 5′-UTR or 147-bp 3′-UTR of TbMCU . To express the ectopic copy of TbMCU, the inducible expression construct pLew100 ( TbMCU-HA ) was generated as described above. The resistance gene cassettes and Not I-linearized pLew100( TbMCU-HA ) (~10 μg) were introduced into T. brucei BSF SM cells by nucleofection using program X-001 and Amaxa Human T-solution following the manufacturer’s instructions. After nucleofection, clones were obtained by limiting dilution and antibiotic selection (2.5 μg ml −1 phleomycin, 5 μg ml −1 blasticidin or/and 0.1 μg ml −1 puromycin). The correct gene replacement or integration in the genome was confirmed by PCR analysis ( Supplementary Fig. S3 ), followed by Southern blot analysis. TbMCU conditional KO BSF mutants were maintained in HMI-9 with 1 μg ml −1 tetracycline, 2.5 μg ml −1 G418 and 5 μg ml −1 blasticidin. To remove tetracycline and shut down expression of ectopic TbMCU , trypanosomes were washed twice and resuspended in culture medium lacking tetracycline. Ca 2+ uptake by digitonin-permeabilized T. brucei The uptake of Ca 2+ by permeabilized T. brucei was assayed by fluorescence measurements at 28 °C using Calcium Green-5N. For PCF, trypanosome cells were collected by centrifugation at 1,000 g for 7 min and washed twice with cold buffer A with glucose, which contained 116 mM NaCl, 5.4 mM KCl, 0.8 mM MgSO 4 , 5.5 mM D -glucose and 50 mM HEPES at pH7.0. PCF cells were resuspended to a final density of 1 × 10 9 cells per ml in the buffer A with glucose and kept on ice. For BSF, trypanosome cells were collected by centrifugation at 1,000 g for 7 min and washed twice with cold separation buffer, which contained 44 mM NaCl, 55 mM D -glucose, 57 mM Na 2 HPO 4 and 3 mM KH 2 PO 4 at pH 8.0. BSF trypanosomes were resuspended to a density of 2 × 10 7 cells per ml in the separation buffer and kept on ice. Before each experiment, a 10-ml aliquot of the BSF cells was concentrated to 50-μl by centrifugation at 1,600 g at room temperature for 3 min. A 50-μl aliquot of PCF (5 × 10 7 cells) or BSF (2 × 10 8 cells) of the cell suspension was added to the reaction buffer (125 mM sucrose, 65 mM KCl, 10 mM HEPES–KOH buffer, pH 7.2, 1 mM MgCl 2 , 2.5 mM potassium phosphate; 2.45 ml) containing 1 μM Calcium Green-5N and the reagents indicated in the figure legends. Ca 2+ uptake by the cells was initiated by the addition of 50 μM digitonin (for PCF) or 40 μM digitonin (for BSF). Fluorescence changes were monitored in a F-4500 fluorescence spectrophotometer (Hitachi) with excitation at 490 nm and emission at 525 nm. Permeabilized cells grown in the presence of tetracycline under the assay conditions used did not show any fluorescence (excitation at 390 nm and emission at 400–650 nm) that could be attributed to tetracycline or its complexes. Mitochondrial membrane potential and phosphorylation Estimation of mitochondrial membrane potential in situ was done spectrofluorometrically using the indicating dye safranine [28] . T. brucei PCF and BSF trypanosomes were incubated at 28 °C in the media described in the figure legends. Fluorescence changes were monitored on a Hitachi 4500 spectrofluorometer (excitation=496 nm; emission=586 nm). Cytoplasmic and mitochondrial Ca 2+ concentrations T. brucei PCF cells were collected by centrifugation and suspended in 5 ml buffer A with glucose containing 2 μM Rhod-2 AM and 0.02% Pluronic F127. After incubation at 27 °C for 50 min in the dark with gentle shaking, cells loaded with Rhod-2 dye were washed and then re-loaded with 5 μM Fluo-4 AM for additional 30 min at 27 °C, followed by an additional 10-min incubation in a dye-free buffer A with glucose. Cells were resuspended to a final density of 1 × 10 9 cells per ml in buffer A with glucose and kept on ice. A 100-μl aliquot (1 × 10 8 cells) of the cell suspension was added to the 1.9-ml reaction buffer. The cytoplasmic and mitochondrial Ca 2+ concentration of cells was monitored in a fluorometer with excitation at 552 nm and emission at 581 nm for Rhod-2 and excitation at 494 nm and emission at 516 nm for Fluo-4, respectively. Fluorescence imaging of [Ca 2+ ] m was carried out by using an Olympus IX-71 inverted fluorescence microscope with a Photometrix CoolSnap HQ charge-coupled device camera driven by DeltaVision software. Mitochondrial oxidative stress Mitochondrial ROS production was measured during the exposure of PCF trypanosomes to digitonin in the presence or absence of Ca 2+ using the fluorescent, mitochondrially targeted probe MitoSOX Red (Invitrogen) as described [57] with some modifications. PCF trypanosomes (2.5 × 10 8 cells per ml) were loaded with 5 μM MitoSOX Red in buffer A with glucose for 10 min at 27 °C and washed once with the same buffer. Cells were resuspended to a final density of 1 × 10 9 cells per ml in the buffer A with glucose and kept on ice. A 100-μl aliquot (1 × 10 8 cells) of the cell suspension was added to the reaction buffer with or without 0.4 mM Ca 2+ and the reagents indicated in the figure legends. The reaction was initiated by the addition of 50 μM digitonin. Fluorescence changes were monitored in a fluorometer with excitation at 510 nm and emission at 580 nm. Adenine nucleotide levels TbMCU RNAi PCF trypanosomes were cultivated in SDM-79 for 4 days with or without tetracycline or in a glucose-depleted medium (SDM-80) containing 5.2 mM L -proline [51] for 2 days in the absence or presence of tetracycline after a 2-day culture in SDM-79 with or without tetracycline. Cells were harvested and washed once with cold buffer A. The cells grown for 4 days in SDM-79 medium were further incubated in buffer A with or without glucose for 1 h at room temperature. After washing or incubation, 1 × 10 8 cells per treatment were centrifuged and resuspended in 100 μl of buffer A, and then lysed on ice for 30 min by addition of 300 μl of 0.5 M HClO 4 . The lysates were neutralized (pH 6.5) by addition of ~150 μl of 0.72 M KOH/0.6 M KHCO 3 . ATP, ADP and AMP in extracted samples were quantified by a luciferin–luciferase bioluminescence assay in a luminometer as described [67] , [68] with some modifications. We used an ATP Determination Kit (Invitrogen) according to the manufacturer’s instructions with adenylate kinase and/or nucleoside-diphosphate kinase (NDK; Sigma). To determine the amount of adenine nucleotides, four measurements were taken of three different reactions for each sample by end point determination of the ATP concentration: one reaction without addition of any ATP-generating enzyme (for ATP), another reaction adding NDK (for ATP+ADP) and the third reaction adding both adenylate kinase and NDK (for ATP+ADP+AMP). The amount of ADP was obtained by subtracting the ATP value from the (ATP+ADP) value and the amount of AMP was calculated from the difference between the (ATP+ADP+AMP) content and the (ATP+ADP) content. Autophagy assay Autophagosome formation in PCF trypanosomes grown in SDM-79 or SDM-80 media, as described above, was estimated by using the autophagy marker TbATG8.2 exactly as described [31] . Effects of RNAi of TbMCU on autophagosome formation were analysed by immunofluorescence microscopy and western blotting using anti- Tc ATG8.2 antibody as described above. Enzyme assays PDH activity was assayed by using a spectrophotometric method as described [69] with some modifications. Briefly, midlog phase PCF and BSF trypanosomes (~2 × 10 8 parasites) were washed in ice-cold PBS with 1% glucose and resuspended in hypotonic lysis buffer (50 mM Tris–HCl, pH 7.4) containing protease inhibitor cocktail. Cells were lysed by freezing and thawing five times using liquid nitrogen (5 min) and a 37-°C water bath (1 min). The protein concentration was determined by using Bio-Rad Bradford assay kit. PDH assays were carried out at 30 °C in the reaction buffer containing 0.3 mM thiamine pyrophosphate, 2 mM NAD + , 2.6 mM cysteine-HCl, 0.12 mM CoA, 0.01 mM CaCl 2 , 0.2 mM MgCl 2 , 5 mM sodium pyruvate and 50 mM MOPS-HCl (pH 7.4). The reaction was initiated by adding 50 μl of cell lysate in a cuvette (light path=1 cm) containing 2.95-ml reaction buffer. The reduction of NAD + was monitored continuously for 5 min by the increase in absorbance ( A ) at 340 nm in a SpectraMax M2 e cuvette reader (Molecular Devices). One unit of enzyme activity is the amount of PDH catalysing the reduction of 1 μmol NAD + per min. Cell death assay T. brucei transgenic PCF trypanosomes overexpressing TbMCU-HA (2 × 10 6 parasites per ml) grown in six-well plates were treated with C2-ceramide (40 μM) for 20 h or H 2 O 2 (100 μM) for 4 h. Cell viability on apoptotic challenge (H 2 O 2 and C2-ceramide) were evaluated by using phase contrast microscopy and further confirmed by using 0.1% Trypan Blue staining. Rounded or straight cells without movement and with Trypan Blue dye staining were defined to be dead cells. The number of viable cells was determined by a haemocytometer using phase contrast microscopy and over 60 fields (including >400 cells) were analysed from each experiment. The percentage of dead cells was obtained by analysing three independent experiments and is expressed as mean±s.d. Statistical analyses are described in Supplementary Methods . In vivo studies Exponentially growing cell lines (WT, RNAi and conditional KO mutants) were washed once in HMI-9 medium without selectable drugs and suspended in the same medium. Eight week-old female Balb/c mice (5–10 per group) were infected with a single intraperitoneal injection of 2 × 10 4 BSF trypanosomes in 0.2 ml HMI-9 medium. For the RNAi and conditional KO mutants, a single inoculum of non-induced trypanosomes was used in two sets of mice with one group being given 200 μg ml −1 doxycycline in 5% sucrose in their drinking water, and the other group being supplied with drinking water containing 5% sucrose only. The drinking water with or without doxycycline was provided 3 days before infection, exchanging it every 2–3 days, and continuing throughout the 30-day period. Feeding doxycycline induced downregulation of TbMCU expression in the RNAi parasites while doxycycline induced the expression of ectopic TbMCU in the conditional KO parasites. Animals were fed ad libitum on standard chow. Parasitemia levels were monitored at 2-day intervals after infection [70] . Mice showing impaired health status and/or with a parasite load >10 8 cells per ml of blood were euthanized. This study was carried out in strict accordance with the recommendations in the Guide for the Care and Use of Laboratory Animals of the National Institutes of Health. The animal protocol was approved by the Institutional Animal Care and Use Committee of the University of Georgia. How to cite this article: Huang, G. et al. Essential regulation of cell bioenergetics in Trypanosoma brucei by the mitochondrial calcium uniporter. Nat. Commun. 4:2865 doi: 10.1038/ncomms3865 (2013).